Berry phases and the intrinsic thermal Hall effect in high-temperature cuprate superconductors Bogolyubov quasiparticles move in a practically uniform magnetic field in the vortex state of high-temperature cuprate superconductors. When set in motion by an externally applied heat current, the quasiparticles’ trajectories may bend, causing a temperature gradient perpendicular to the heat current and the applied magnetic field, resulting in the thermal Hall effect. Here we relate this effect to the Berry curvature of quasiparticle magnetic sub-bands, and calculate the dependence of the intrinsic thermal Hall conductivity on superconductor’s temperature, magnetic field and the amplitude of the d-wave pairing. The intrinsic contribution to thermal Hall conductivity displays a rapid onset with increasing temperature, which compares favourably with existing experiments at high magnetic field on the highest purity samples. Because such temperature onset is related to the pairing amplitude, our finding may help to settle a much-debated question of the bulk value of the pairing strength in cuprate superconductors in magnetic field. Low-energy excitations of a superconductor, the Bogolyubov quasiparticles (QPs), are quantum mechanically coherent superpositions of an electron and its absence, the hole. Therefore, QPs do not carry a fixed electrical charge. In the vortex state of extreme type-II superconductors, such as high transition temperature cuprates, the externally applied magnetic field H penetrates the sample in the form of flux tubes, whose width is set by the material-specific parameter named penetration depth. For essentially the entire range of H fields applied in a typical experiment, the cuprates’ penetration depth is much larger than the inter-vortex separation, the latter being set by the magnetic length . Here H is the magnitude of the applied field, h the Planck’s constant, c the speed of light in vacuum and e the electron charge. Therefore, the QPs move in a practically uniform magnetic (induction) field B . Suppose that QPs are set in motion by applying a small energy current j E whose direction is perpendicular to H . If the resulting net flow velocity of QPs is deflected preferentially to one side, their energy is deposited at the corresponding edge of the sample, causing a transverse gradient of superconductor’s temperature T , that is, a non-zero off-diagonal component of the Fourier law or, equivalently, the thermal Hall effect. Relatedly, among the best established physical properties of cuprate superconductors in the vortex state is the increase of the low T specific heat when the H -field is applied perpendicular to the CuO 2 planes. This effect was predicted by Volovik [1] based on a semiclassical analysis of the QP motion in the vortex state of a wave superconductor. Although Volovik’s semiclassical approximation successfully captures the overall increase of the QP density of states, a full quantum mechanical solution is needed to calculate the QPs’ contribution to the thermal Hall conductivity, κ xy , because, as discussed below, this quantity is related to the non-trivial topological structure of the QP wavefunctions. The thermal Hall effect has been reported experimentally in (slightly hole overdoped) YBa 2 Cu 3 O 6.99 samples by Ong and collaborators [2] , and by Zeini and collaborators [3] . The measurements [2] extend up to 15 T, and down to the lowest T of 12.5 K. κ xy is positive (hole-like), and decreases with decreasing T . However, linear extrapolation to T →0 would yield a finite negative value of κ xy , which is unphysical because κ xy / T would diverge in such a limit. Rather, the data [2] at the highest fields are consistent with κ xy being very small below T onset ~7 K, followed by a rapid increase at T onset with an almost linear T dependence at higher T . The initial theoretical approach [4] was based on a continuum model with the linearized dispersion relation in the vicinity of the nodal Dirac points of the superconductor’s spectrum at H =0. In ref. 4 , the Kubo formula was used to argue for the scaling form κ xy ~ T 2 F ( k B Tℓ H / ħv ), where F has been hitherto an undetermined scaling function, k B is the Boltzman constant, , and p F and v F are the nodal Fermi momentum and velocity, respectively. The parameter Δ quantifies the energy of the d-wave pairing amplitude. Based on the same linearized continuum model, it was also argued [5] that the QP Dirac spectrum in the vortex state acquires a mini-gap, which grows linearly with H , and that with n =0 or ±2. Unfortunately, the linearized approximation, on which these conclusions rest, has been found to be problematic. Within the linearized approximation, the QP spectrum is not [6] , [7] invariant under the large (singular) gauge transformations [8] , [9] , which were being employed in the calculations [5] of κ xy . Because such large gauge invariance must hold, the validity of the results has been in doubt. A tight-binding lattice regularization was found to remove such problems [6] . The initial model calculation [10] of κ xy using such regularization was limited to unrealistically large values of H , indeed finding that for a space inversion symmetric vortex lattice, the QP spectrum is generally gapped and that , albeit the values of n ranged from −2 to 12. Subsequent index theoretic results [11] , limited to densities very close to one electron per lattice site, found commensuration-based mini-gap oscillations with n =0, ±4. Finally, using the linearized approximation and a number of drastic simplifying assumptions, the weak field was argued to be due to thermally excited nodal QPs, scattering primarily from impurities, with a small skew component due to vortices [12] . In this work, we present results of an extensive numerical calculation providing detailed T , H and Δ dependence of the intrinsic contribution to κ xy . Because j E is perpendicular to the thermal Hall gradient, the thermal Hall effect does not contribute to entropy production, . Therefore, there is an intrinsic contribution to the corresponding non-dissipative transport coefficient, independent of the details of the relaxation processes, which return the system to equilibrium. Such an intrinsic contribution to κ xy , which we expect to dominate in the clean limit, is a direct consequence of the QP wavefunctions acquiring a non-trivial Berry curvature [13] upon adiabatic changes of the vortex crystal momentum [10] , k . We thus calculate κ xy using the tight-binding regularization for a d-wave superconductor—whose H =0 pairing function is 2Δ(cos k x −cos k y )—and for a variety of H values and vortex lattice geometries. Our main finding is that, when properly rescaled by its value in the normal state, which is also assumed to be in the clean limit, κ xy does not depend on the structure of the vortex lattice or H , assuming of course that H is not large enough to destroy superconductivity. When T is reported in units of Δ, here varied independently of H , the important dimensionless quantity determining the T dependence of κ xy is the anisotropy of the dispersion near the gap node, α D , and even here the dependence is weak. The scaling collapse thus attained clearly displays the rapid temperature onset at a small fraction of Δ followed by an almost linear T dependence. This finding may establish measurements of κ xy as a means to obtain bulk spectroscopic information about high-temperature superconductors, and provide an avenue for resolving the pressing question regarding the overall strength of Cooper pairing in high magnetic field [14] . The QP density of states and the κ xy scaling We motivate the description of the details of the model and its analysis by first showing the main results, which were obtained using the Hamiltonian in equation (1). 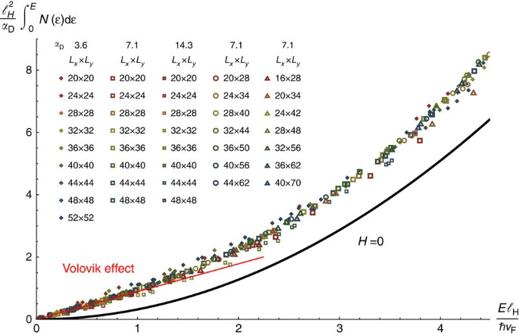Figure 1: Quasiparticle (QP) density of states scaling. Integrated QP density of states (IDOSs) per area versus QP energy for a number of magnetic fields, vortex lattice geometries and the nodal dispersion anisotropiesαD=vF/vΔof 3.6, 7.1 and 14.3. The vertical axis, IDOS, is rescaled by the square of the magnetic length,, and by 1/αD. The horizontal (energy) axisEis rescaled byħvF/ℓH, wherevFis the Fermi velocity at the node. The solid black curve is the IDOS forH=0, which grows as ~E2for smallE, graphed assuming increasingly smallEand increasingly largeℓH, such thatEℓHis finite; only the quadratic term in the Taylor expansion of IDOS inEsurvives in this limit. The Volovik effect corresponds to IDOS vanishing linearly withE(solid red line), with slope of ≈0.9. For orientation, takinga=3.8 Å andLx=Ly=32aresults inH≈28 T, becauseHLxLya2=hc/e. Converting to the lowT-specific heat per mole of formula unit gives. Figure 1 shows the QP density of states per area at energy , , integrated from up to . The reason for plotting the integrated density of states (IDOSs), as opposed to , is that the QP spectrum is described by a large number of magnetic sub-bands whose number grows with decreasing magnetic field as 1/ H . Being in two space dimensions, each one of the sub-bands harbours at least one van Hove singularity with a logarithmic divergence of . Thus, plotting the contribution from each sub-band to leads to large variations of the resulting dependence, obscuring the main physical effect. On the other hand, the IDOS simply counts the number of eigenstates between 0 and E , which is smoother, and lends itself more readily to physical insight. Indeed, the H -induced increase in the number of states at low energy is clearly seen on the scaling plot marked by various symbols in Fig. 1 , when compared with the result at H =0 shown as the solid black line. At H =0, at small , and therefore ; this can be graphed on the scaling plot assuming increasingly small E and increasingly large ℓ H , such that Eℓ H is finite, because only the quadratic term in the Taylor expansion of IDOS in E survives in this limit. The low-energy portion of the spectrum is thus seen to obey Simon and Lee scaling [4] to a very good approximation. Furthermore, Volovik’s result [1] , , appears as the linear dependence of the scaled IDOS marked by the red line. The key point here is that, on average, the external magnetic field increases the number of QP states at low energy. The next question that we address is their contribution to the intrinsic κ xy . Figure 1: Quasiparticle (QP) density of states scaling. Integrated QP density of states (IDOSs) per area versus QP energy for a number of magnetic fields, vortex lattice geometries and the nodal dispersion anisotropies α D = v F / v Δ of 3.6, 7.1 and 14.3. The vertical axis, IDOS, is rescaled by the square of the magnetic length, , and by 1/ α D . The horizontal (energy) axis E is rescaled by ħv F / ℓ H , where v F is the Fermi velocity at the node. The solid black curve is the IDOS for H =0, which grows as ~ E 2 for small E , graphed assuming increasingly small E and increasingly large ℓ H , such that Eℓ H is finite; only the quadratic term in the Taylor expansion of IDOS in E survives in this limit. The Volovik effect corresponds to IDOS vanishing linearly with E (solid red line), with slope of ≈0.9. For orientation, taking a =3.8 Å and L x = L y =32 a results in H ≈28 T, because HL x L y a 2 = hc / e . Converting to the low T -specific heat per mole of formula unit gives . Full size image The principal result of this paper is shown in Fig. 2 . κ xy was calculated for several values of H and vortex lattice geometries as indicated in the legend by the values of the dimensions of the magnetic unit cell L x × L y , given in the units of the underlying tight-binding lattice spacing, a . We made sure that the values of L x and L y were chosen to be sufficiently large so that the low-energy IDOS collapses on the scaling curve shown in the Fig. 1 . Within our model, the normal state value, κ xy ( T , 0, H ), is also computed in the clean limit: in the low T regime where it is T linear, κ xy ( T , 0, H ) scales as 1/ H . Such dependence on T and H also follows from the clean free Fermion limit given by the Wiedemann–Franz relation , where the electrical Hall conductivity . The plot of the ratio κ xy ( T , Δ, H )/ κ xy ( T , 0, H ) versus T /Δ, in the regime where κ xy ( T , 0, H ) is T linear, is shown by the solid lines for a fixed value of H and the square vortex lattice 28 a × 28 a , and for six different values of the nodal dispersion anisotropy α D = v F / v Δ indicated next to each solid line. In addition, for fixed α D =7.1, the κ xy ratio is shown using various symbols for different values of H and vortex lattice geometries, as indicated by the three columns in the legend. The quality of the collapse for α D =7.1 is representative of the scaling at different values of α D , which we do not show to avoid clutter. The κ xy ratio is seen to collapse quite well onto a single curve for each value of the nodal velocity anisotropy, α D , and to approach 1 with increasing k B T /Δ, independent of the vortex lattice geometry; here k B is the Boltzmann constant. Moreover, the rapid T onset occurs at the value of T set predominantly by (a fraction of) the value of Δ, with a weak residual dependence on α D . This is followed by the regime of approximately T linear dependence with a negative extrapolated vertical intercept. These theoretical results indicate that experimental measurements of the onset T for fixed values of H can therefore be translated to the H dependence of the maximum magnitude of the d-wave Cooper pair amplitude. This would provide highly desirable information on the suppression (or lack thereof) of the superconducting order parameter amplitude by the external magnetic field. 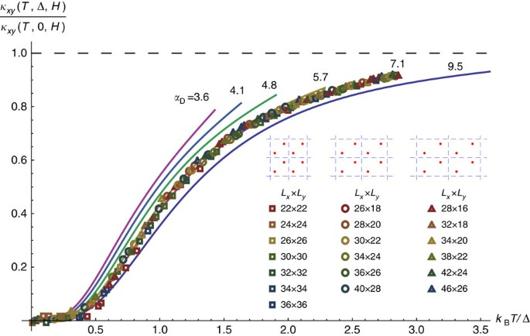Figure 2: Thermal Hall conductivity scaling. Intrinsic contribution to the thermal Hall conductivityκxyin the vortex state ofwave superconductor, with the zero field (H=0) pairing function 2Δ(coskxa−coskya), versus the ratio of temperature and Δ. The vertical axis is rescaled by the clean normal state valueκxy(T, Δ=0,H)~T/H. The dimensions of the magnetic unit cell,Lx×Ly, are given in the units of the underlying tight-binding lattice spacinga. The solid lines are calculated for a fixed value ofHfor the square vortex lattice 28a× 28a, and for six different values of the nodal dispersion anisotropyαD=vF/vΔindicated next to each solid line. In addition, for fixedαD=7.1, theκxyratio is shown using various symbols for different magnetic field values and vortex lattice geometries, as indicated by the three columns in the legend. For fixed Δ, the results collapse well onto a single scaling curve, exhibiting a rapid increase at a small value ofkBT/Δ. The scaling functions display an additional weak dependence onαD. Figure 2: Thermal Hall conductivity scaling. Intrinsic contribution to the thermal Hall conductivity κ xy in the vortex state of wave superconductor, with the zero field ( H =0) pairing function 2Δ(cos k x a −cos k y a ), versus the ratio of temperature and Δ. The vertical axis is rescaled by the clean normal state value κ xy ( T , Δ=0, H )~ T / H . The dimensions of the magnetic unit cell, L x × L y , are given in the units of the underlying tight-binding lattice spacing a . The solid lines are calculated for a fixed value of H for the square vortex lattice 28 a × 28 a , and for six different values of the nodal dispersion anisotropy α D = v F / v Δ indicated next to each solid line. In addition, for fixed α D =7.1, the κ xy ratio is shown using various symbols for different magnetic field values and vortex lattice geometries, as indicated by the three columns in the legend. For fixed Δ, the results collapse well onto a single scaling curve, exhibiting a rapid increase at a small value of k B T /Δ. The scaling functions display an additional weak dependence on α D . Full size image The model Hamiltonian We work on a two-dimensional square lattice of spacing a —that we set to unity—and H perpendicular to it. Our tight-binding Hamiltonian describing excitations of the d-wave superconductor in the vortex state is This model has been discussed extensively elsewhere [6] , [11] , [15] : c r , σ is the electron annihilation operator, the sum over the spin projection σ =↑ or ↓ in the first and the last terms is implicit, and H.c. stands for Hermitian conjugation. The chemical potential and the Zeeman coupling enter via μ ↑(↓) = μ ± h Z . The magnetic flux Φ through an elementary plaquette enters the Peierls factors as and , where φ 0 = hc / e . The ansatz for the pairing term is , with the d-wave amplitude and the line integral is along the nearest neighbour link. Vortex positions, r j , residing in the centres of (some of) the elementary plaquettes, enter the pairing term through θ ( r ), which is chosen to be the solution of the (continuum) London’s equations , ∇ · ∇ θ ( r )=0. The closed form solution for θ ( r ) can be found in the Methods section. Vortices are arranged within the magnetic unit cell as shown in the legend of Fig. 2 . Each L x × L y magnetic unit cell—aligned with the tight-binding lattice formed by the 1 × 1 elementary plaquettes—is threaded by magnetic flux hc / e and contains a pair of vortices. Performing the singular gauge transformation [6] , [8] , [11] turns the hopping and the pairing terms in periodic with periodicity L x and L y , allowing us to use the Bloch theorem [6] , [8] , [11] . As such, we perform the (unitary) particle-hole transformation by letting , where is periodic in r → r + R , N uc is the number of unit cells, and, within the sum, k lies within the magnetic Brillouin zone, − π / L x,y ≤ k x,y < π / L x,y . In terms of the transformed operators (momentarily suppressing ’s argument k ): where the spin preserving hopping amplitudes are , the spin flipping hopping amplitudes are . In the sum, r is limited to the L x × L y unit cell, and the sum over the two spin projections is implicit in the term containing . Further details, including the treatment of the branch-cuts in the hopping amplitudes, are provided in the Methods section. Equation (2) has the form of a Hamiltonian for a fictitious semiconductor with spin-orbit coupling. Although the time-reversal symmetry is explicitly broken in the equation (2), the magnetic vector potential does not couple minimally in all the complex hopping parameters [8] , and as such there is no Lorentz force on ’s. By direct analogy with the anomalous Hall effect [16] in metals, any intrinsic κ xy is therefore driven by Berry phase mechanisms. The Heisenberg equations of motion, , define the single particle Bloch Hamiltonian, , whose discrete eigenvalues, E m ( k ), and eigenstates, | m k ›, are labelled by a discrete magnetic sub-band index, m . For H ≠0 and Δ=0, the model in equation (1) reduces to the well-known square lattice Hofstadter ‘butterfly’ problem [17] , with flux per plaquette , where . Momentarily ignoring the twofold spin degeneracy, the Chern integers l r , determining the electrical Hall conductivity associated with M filled sub-bands, obey the Diophantine equation [18] , [19] , , where s is an integer and where l r is subject to the restriction . Solving for l r we find that [19] (for even ) each of the lowest, and each of the highest, sub-bands carries the Chern number l r − l r–1 =+1. In addition, there is a pair of touching sub-bands straddling the midline of the energy spectrum, which carries the (large) Chern number , equally divided between the two anomalous sub-bands [19] . Near the H =0 band extrema, the (Landau) energy gaps between the magnetic sub-bands are , because there the H =0 energy dispersion is parabolic. For H =0 and Δ≠0, the QP spectrum of is , with and Δ( k )=2Δ(cos k x –cos k y ). There are four gapless Dirac points in the first Brillouin zone, with the velocity anisotropy α D = v F / v Δ = t /Δ, which dominate the low-temperature thermodynamics. Thus, the pairing term in mixes sub-bands near the Fermi level. In the physically relevant situation, each of these magnetic sub-bands mixed by Δ carries a unit Chern number, thus resembling Landau levels of a continuum problem. Moreover, the number of such occupied sub-bands should be large compared with . Therefore, we choose to set μ =2 t , corresponding to ≈0.37 holes per site. With this choice the pairing term does not mix the anomalous band with the large Chern number, while at the same time the pairing term remains small compared with the Fermi energy. We now turn to H ≠0 and Δ≠0. In the semiclassical approximation of Volovik [1] , the spatially varying phase θ ( r ) induces a finite zero-energy density of states, , which scales as . More generally, the scaling expected [4] , [8] from the approximate Dirac model is . As shown in Fig. 1 , up to small variations [15] , we indeed recover this scaling in our model when . The IDOSs per area, per spin, per layer is seen to follow the scaling , where for with b ≈0.9 and for , regardless of the shape of the vortex lattice, as long as α D ≳ 3. This implies that the low- T specific heat per mol of formula unit is . For example, in YBa 2 Cu 3 O 7−δ , n layers =2 because there are two CuO 2 layers per unit cell whose Area[ nm 2 ]≈0.149. Intrinsic contribution to κ xy It has long been known that for H ≠0 the thermal transport coefficients cannot be calculated using the Kubo formula alone [10] , [20] , [21] , [22] , [23] . Rather, κ xy is given by [10] , [22] where and The double sum over m and n is to be performed subject to the stated constraint on the eigenenergy. It is well known that , where Ω m ( ξ ) is the integral over the Berry curvature of the m th magnetic sub-band over the parts of the magnetic Brillouin zone, which are below the energy ξ . If the QP sub-band is fully occupied then the integral over the Berry curvature is the first Chern number, which is to say, an integer [10] , [18] . Our main result is shown in Fig. 2 . The rapid onset of κ xy with increasing T can be understood from the ξ dependence of and the formula in equation (3). The quantity , shown in Fig. 3 , has a simple physical interpretation: it is proportional to the QP contribution to the T =0 spin Hall conductivity [10] if all the QP sub-bands below the energy ξ are occupied. In addition, for Δ=0 it can be related to the usual electrical Hall conductivity due to, say, spin up electrons only, at the Fermi energy E F . Indeed, for Δ=0, , where the first term corresponds to the contribution of the spin-up electrons and the second to the spin-down holes moving in the opposite magnetic field. We see that for Δ=0, the quantity ξ can be interpreted as a fictitious Zeeman energy splitting. Therefore, the loss of the total Chern number in the minority band is largely compensated by the gain in the majority band, and for Δ=0, is essentially independent of ξ . For a range of ξ ’s near zero, its value is approximately 2 l r , that is to say the solution of the mentioned Diophantine equation determining the normal state electrical conductivity at μ (see 1/ α D =0 curve in the Fig. 3 for small ξ ). This is expected, as an analogous formula to equation (3) holds in the normal state as well [22] , in which case it relates the electrical Hall conductivity to the thermal Hall conductivity. 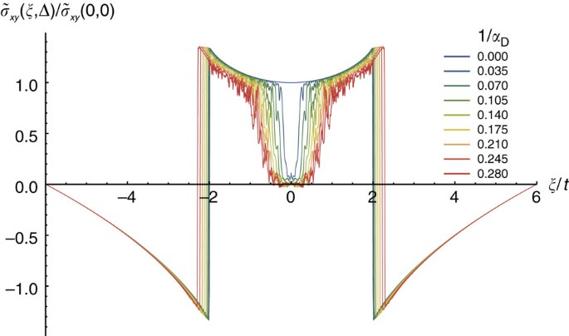Figure 3: Integrated Berry curvature. Energy dependence of the momentum space integrated Berry curvature, summed over all Bogolyubov quasiparticle (QP) states that are below the energyξ. Hereis proportional to theT=0 spin Hall conductivity when all the QP bands belowξare occupied (see equation 4), and plotted for various values of the nodal dispersion anisotropyαD=vF/vΔ. The vertical axis is rescaled by the by the normal state value atξ=0, namely. The horizontal axis is rescaled by the tight-binding hopping amplitudet. The curves graphed here were calculated for a square vortex lattice withLx=Ly=28a. The thermal Hall conductivityκxyis obtained fromusing the equation (3). Figure 3: Integrated Berry curvature. Energy dependence of the momentum space integrated Berry curvature, summed over all Bogolyubov quasiparticle (QP) states that are below the energy ξ . Here is proportional to the T =0 spin Hall conductivity when all the QP bands below ξ are occupied (see equation 4), and plotted for various values of the nodal dispersion anisotropy α D = v F / v Δ . The vertical axis is rescaled by the by the normal state value at ξ =0, namely . The horizontal axis is rescaled by the tight-binding hopping amplitude t . The curves graphed here were calculated for a square vortex lattice with L x = L y =28 a . The thermal Hall conductivity κ xy is obtained from using the equation (3). Full size image For Δ≠0, the still reaches the value ≈2 l r , which is of order , when . This happens because for ξ large compared with Δ, the contribution to the Chern numbers comes predominantly from the QP bands, which are weakly affected by the pairing term. On the other hand, when , then becomes small, non-universal and its value oscillates around zero. This trend is displayed in Fig. 3 , where the ξ dependence of , rescaled by its value in the normal state and ξ =0, is shown for various values of 1/ α D =Δ/ t . Such a precipitous drop near ξ =0 is a consequence of the QP states near zero energy being an almost equal superposition of the electron and a hole, ridding the sub-bands of the Berry curvature. It is fully consistent with the previous result [11] where the value of , small compared with , was obtained near μ =0. Convolving such ξ dependence of with the thermal factor in equation (3) at low T results in a vanishingly small κ xy . As the temperature increases, the thermal function broadens, and the rapid increase of with increasing ξ is mirrored by the rapid increase of κ xy with increasing T . We restrict in Fig. 2 , guaranteeing that in the normal state (Δ=0), κ xy is linear in T . The H dependence follows readily from the above discussion as well. Since for , , we find that the H dependence of κ xy (Δ≠0) is determined by the H dependence of κ xy (Δ=0)~1/ H . We also find the dependence of κ xy on the Zeeman coupling, h Z , to be barely observable when . This is due to the fact that, with the Zeeman term, we convolve the average of instead of . For any , the main effect of the averaging is to smear the fluctuations in , whereas the overall shape of the curve remains essentially unchanged. Similarly, we find negligible dependence on the size of the vortex core as long as it is small compared with the inter-vortex separation. The importance and the novelty of our results stem from the role that the overall d-wave pairing strength, Δ, plays in determining the temperature scale at which κ xy rapidly increases from a negligibly small value at low T . It may therefore serve as an important probe of the cuprate superconductors, and perhaps other materials as well, and provide a means of measuring Δ via a bulk transport measurement. In the clean limit, this method could become very attractive as, unlike the specific heat, κ xy is not contaminated by other degrees, notably phonons which are electrically neutral and whose trajectories do not bend by the Lorentz force. Moreover, the measurement can be performed at a high magnetic field, which can be held constant, and the onset temperature measured by sweeping T . It would be very interesting to measure the H dependence of the onset temperature starting from the small values of H well inside the superconducting state all the way to (and past) the resistive field, H irr , which marks the transition from the superconductor to a fascinating, and presently poorly understood, resistive low T state of electronic matter. Is the onset temperature gradually suppressed by H , making it vanish in some smooth fashion at the H irr , does it remain finite above H irr , or does it collapse discontinuously? Experimental answers to these questions would provide important clues as to the nature of the resistive high field, low temperature, state. Determination of the phase field The closed form solution of London’s equations for the pairing phase field with the periodic arrangement of vortices is Here, using the complex notation, z= x + iy , and the summation over j accounts for the position of the vortices within the magnetic unit cell z j = x j + iy j , of which there are two for the configurations shown in the legend of Fig. 2 . Therefore, in our case n V =2. σ ( z – z j ; ω , ω ′) is the Weierstrass σ function with periods ω = L x and ω ′= iL y . Constants γ and v 0 are determined by the boundary conditions. In order to ensure that the superfluid velocity satisfies periodic boundary conditions, we must have , where ζ ( z ; ω , ω ′) is the Weierstrass ζ function. The former boundary condition ensures that the hopping amplitudes in equation (2) are periodic. For square lattices, γ =0. In order for the spatial average of the supercurrent to vanish, we must have . Phase factors involving θ ( r )/2 should be handled with care because of the sign ambiguity associated with taking the square-root. First, we (periodically) connect vortices pairwise within each magnetic unit cell with branch-cuts [11] . For the spin preserving hopping amplitudes in equation (2), we choose the signs so that , where the line integral is over the nearest neighbour link. The periodic factor on each nearest neighbour link except the ones crossing the branch cut where . This identity follows readily from considering products over the links forming closed clockwise loops around elementary plaquettes. The left hand side must give +1 around each loop because it consists of a product of complex numbers with unit magnitude on each site. On the other hand, the (link) term on the right hand side gives −1 if the plaquette contains a vortex and +1 if it does not, because in the first case and 0 in the second. Also note that . In practice, for the values of L x and L y considered in this work, we found that within the first magnetic unit cell, , which is convenient because only site variables are involved. Similarly, for the spin flipping hopping amplitudes, . We used standard numerical methods for finding all eigenvectors and eigenvalues of a complex Hermitian matrix to which the Hamiltonian presented in equation (2) can be straightforwardly brought. Owing to the specific arrangement of vortices, the Hamiltonian in equation (2) possesses symmetries, which consist of either point group operations alone or point group operations combined with the time reversal and/or gauge transformations. These symmetries are reflected in the solution for the phase field, equation (5), and thereby in the hopping amplitudes. From there one can show that the single particle Bloch Hamiltonians and , defined below the equation (2), are related by a unitary or an anti-unitary operation, when k and k ′ are symmetry related. It is not necessary to take advantage of these symmetries, but the numerical calculation is faster by about an order of magnitude if this is done. Numerical evaluation of The expression in equation (4) can be written as , with being the Berry curvature at k summed over all states that are below ξ at k . The matrix elements are . The calculation of requires computationally costly operations, diagonalization of large matrices whose dimension is and summation over a large number of states. Our strategy to effectively calculate is to start with the observation that for fixed k , is a constant as a function of ξ , unless ξ coincides with one of the Hamiltonian eigenvalues, say E l ; there exhibits a jump. This property allows us to create an ordered lookup table where we store pairs of values , that is, the list of increasing eigenvalues and corresponding ’s at ξ ’s just above each eigenvalue. Once the lookup table has been created, finding requires a search for the highest E l < ξ in the lookup table and reading off the corresponding . Given that the table is ordered, the complexity of such an operation is , which is fast. The computational cost of the diagonalization of the Hamiltonian at k is because we need the entire spectrum as well as all the eigenstates. Naively, in the equation (6) contains the summation over two indices, m and n , and both sums have terms, unless ξ is close to the bottom or the top of the H =0 tight-binding band. Furthermore, finding each would seem to require summing terms. In total, these estimates imply that the creation of a lookup table has the computational complexity of . We reduce the complexity to using several observations. First, the difference between two adjacent ’s in the lookup table is given by Thus, we are left with only terms to sum over. Therefore, if we build the lookup table by recursively adding the result of equation (7) to to obtain , remembering that for ξ < E 1 , then we sum only terms for each lookup table entry instead of . This leads to improvement over the original double summation formula, equation (6). Second, we observe that for each k , are sparse matrices, each having only non-zero elements. This follows from the fact that they derive from the single-particle Hamiltonian , which is a sparse matrix. The computation of therefore requires a summation of only terms, thereby improving the computational time by another factor. The computation of ’s can be further optimized by noticing that, once l is fixed, we can find , store the two vectors for μ = x , y and use them to compute and faster. Overall, we find that the computational complexity of the lookup table creation is if equation (4) is used together with these improvements. From the expression , we see that can be approximated and calculated by expressing it as a Riemann sum, where the integration domain, in our case the magnetic BZ (or fraction thereof if symmetries are used), is partitioned into s non-overlapping patches, each with area A i . For each patch, the Berry curvature is calculated at some point k i within that patch. We partitioned the integration domain using an adaptive mesh integration method. This method starts with a coarse mesh of k points and then refines the mesh by increasing the density of k points in the patches where the absolute errors are the largest. In this manner, the overall error is minimized using the fewest number, s , of k points where is calculated. How to cite this article: Cvetkovic, V. & Vafek, O. Berry phases and the intrinsic thermal Hall effect in high-temperature cuprate superconductors. Nat. Commun . 6:6518 doi: 10.1038/ncomms7518 (2015).